Terrestrial selenium distribution in China is potentially linked to monsoonal climate The prevalence of terrestrial environments low in the essential trace element selenium (Se) results in large-scale Se deficiency worldwide. However, the underlying processes leading to Se-depleted environments have remained elusive. Here we show that over the last 6.8 million years (Ma) climatic factors have played a key role in the Se distribution in loess–paleosol sequences in the Chinese Loess Plateau (CLP), which lies in a severely Se-depleted region with a history of Se deficiency-related diseases. We use a combination of geochemical and paleoclimate data to demonstrate that during interglacial periods between 2.30 and 0.16 Ma, variations in the Se concentration in the CLP are potentially related to variability in Se input via East Asian monsoon-derived precipitation. Our results identify precipitation as an important controlling factor of Se distribution in monsoonal China. We suggest that atmospheric Se inputs via precipitation could also play an important role in other regions worldwide. Selenium (Se) is an essential trace element for human health [1] . Foodstuffs are an important source of Se to humans [2] ; however, Se intake worldwide is highly variable due to its heterogeneous distribution in agricultural soils and the terrestrial environment in general [1] , [3] . Globally, Se deficiency is a major health problem with estimates of 0.5–1 billion people being affected by low Se intake [4] . The ‘Se-poor belt’ in Central China ( Fig. 1a ) is a clear example of an area in which extremely low soil-Se concentrations correlate with low Se intake and a high prevalence of related diseases such as Kashin–Beck disease, a chronic bone and cartilage disease, and Keshan Disease, a chronic heart disease, both of which primarily affect young children and women of child-bearing age [5] , [6] . 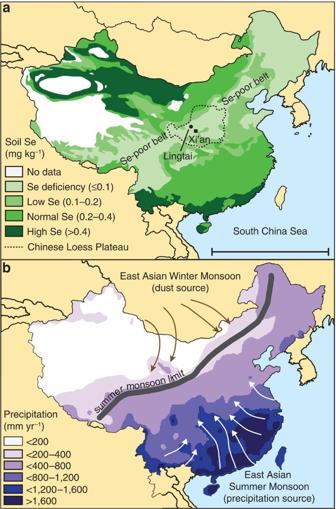Figure 1: Patterns of soil selenium and precipitation in China. (a) Soil selenium distribution5and (b) average precipitation distribution from 1980–2010 (ref.49). The dashed line indicates the extent of the Chinese Loess Plateau and the black circle indicates the studied Lingtai section. The thick grey line indicates the northernmost extent of the East Asian summer monsoon (that is, summer monsoon limit). White arrows indicate dominant weather directions of the East Asian summer monsoon (EASM) and dark brown arrows indicate the main directions of the East Asian winter monsoon (EAWM). Figure 1: Patterns of soil selenium and precipitation in China. ( a ) Soil selenium distribution [5] and ( b ) average precipitation distribution from 1980–2010 (ref. 49 ). The dashed line indicates the extent of the Chinese Loess Plateau and the black circle indicates the studied Lingtai section. The thick grey line indicates the northernmost extent of the East Asian summer monsoon (that is, summer monsoon limit). White arrows indicate dominant weather directions of the East Asian summer monsoon (EASM) and dark brown arrows indicate the main directions of the East Asian winter monsoon (EAWM). Full size image The distribution of Se in the terrestrial environment (for example, soils and crops) is poorly understood. Underlying bedrock geology has traditionally been viewed as the primary source of Se in soils [7] . However, this factor alone cannot explain the large-scale distribution of Se but rather explains localized areas with high soil-Se concentrations, for example, at Enshi, Hubei Province, China, where weathering of carbonaceous black shales has led to very high (up to 60 mg kg −1 ) soil-Se concentrations [8] , [9] . Another source of Se in the terrestrial environment could be the atmosphere, which is an important reservoir in the Se cycle [10] , [11] , [12] , [13] , [14] . The marine environment has been identified as the largest natural source of Se to the atmosphere [12] , [13] , [14] . Se is methylated by marine organisms (for example, coccolithophorids) in the oceans and is released largely as volatilized gaseous dimethyl selenide and dimethyl diselenide [15] , [16] . These gaseous Se species are oxidized within minutes to hours to inorganic species such as Se(0), SeO 2 and H 2 SeO 4 , and are transported through the atmosphere and deposited [17] . Atmospheric Se mass-balance calculations indicate that wet deposition is the dominant mechanism of atmospheric Se deposition and selenite (Se(IV), SeO ) and selenate (Se(VI), SeO ) have been found as the dominant Se species [18] , [19] , [20] . Global Se deposition by precipitation has been estimated to be 35–100 × 10 8 g Se per year compared with 17–24 × 10 8 g Se per year via dry deposition [11] , although these processes are presumably highly dependent on local and regional conditions. Whereas Se has been shown to be enriched in sea spray and precipitation in coastal areas [18] , there has been little evidence indicating long-range transport of Se to inland terrestrial environments. We focus our study on the relationship between precipitation and Se distribution in the Chinese Loess Plateau (CLP, Fig. 1a ), the biggest accumulation of windblown sediments on earth [21] , which lies in the Se-poor belt ( Fig. 1a ). The CLP has a clearly defined and well-documented seasonal precipitation source; the East Asian summer monsoon (EASM, Fig. 1b ). The EASM, carrying moisture from the China Sea, begins moving north in late April to early May, reaches its northernmost extent (that is, summer monsoon limit, see Fig. 1b ) in central China during late July to early August and then subsequently retreats south [22] . Changes in the strength of the EASM over the last 7 million years (Ma) have been recorded in the extensive, alternating deposits of loess (that is, windblown mineral dust) and paleosols that compose the CLP and thus have made it a well-studied continental climate archive [23] , [24] , [25] , [26] , [27] , [28] . Loess layers represent past glacial periods in which the East Asian winter monsoon (EAWM) was particularly strong and large amounts of dust were transported to the CLP from the north-northeast ( Fig. 1b ). Paleosol layers, in contrast, were formed during interglacial periods when the EASM was strengthened, which resulted in increased weathering and paedogenesis [29] . Interestingly, the current summer monsoon limit geographically coincides with the Se-poor belt (compare Fig. 1a,b ). Whereas the high soil-Se concentrations in northwest China ( Fig. 1a ) may be due to enrichment in drier saline-alkaline soils [30] , the similarity between Se soil distribution and precipitation south of the summer monsoon limit is striking (compare Fig. 1a with Fig. 1b ), suggesting that rainfall is an important factor in controlling the Se distribution in this area, which is the most densely populated region of China. The purpose of this study is to investigate the Lingtai loess-red clay sequence ( Fig. 1a ) as a potential long-term environmental archive of atmospheric Se deposition with the objective of understanding how atmospheric Se impacts the terrestrial distribution of Se. We use geochemical and paleoclimate data to show that precipitation has played a key role in the variation of Se in the CLP. The results of our study suggest that soil Se distribution patterns in monsoonal China may be partially explained by precipitation as a source factor. Sources of Se and common trends with global benthic δ 18 O We hypothesize that Se in the CLP has two main sources: the dust associated with the EAWM and the precipitation coming with the EASM. As these are the only sources of Se to the CLP, bedrock weathering can be excluded as a major source of Se. To test our hypothesis, we investigated the relationship between Se and summer and winter monsoon proxies (that is, carbonate content and magnetic susceptibility in paleosols [23] , [31] , [32] , [33] , and mean quartz grain size and dust mass accumulation rate in loess layers [25] , [34] , [35] , respectively) ( Supplementary Fig. 1 ). Our analyses reveal that the Se concentrations in all samples are below the 0.1 mg kg −1 concentration limit under which soils are considered Se deficient [36] . Although average Se levels in loess and paleosols are nearly identical (45 μg kg −1 and 46 μg kg −1 , respectively), we find that during the wetter interglacial periods (paleosols), there are moderate to very strong alternating positive and negative correlations between Se and global benthic δ 18 O ( Fig. 2a ), a paleo-temperature proxy relating to both the EAWM and EASM [24] , [25] , [27] . Based on these correlations, we defined four distinct periods in the paleosols which we analysed further: period I, 2.31–1.56 Ma (Spearman’s correlation coefficient ( ρ )=−0.94, P <0.001); period II, 1.50–1.29 Ma ( ρ =0.82, P =0.058); period III, 1.26–0.83 Ma ( ρ =−0.67, P =0.083); and period IV; 0.78–0.16 Ma ( ρ =0.78, P =0.017). The relationship between Se and the global benthic δ 18 O record is not fully understood and warrants further investigation, nonetheless in these four periods the summer monsoon index (SMI), a proxy for effective precipitation that combines magnetic susceptibility and carbonate content proxies [31] also displays moderate to very strong alternating positive and negative relationships with δ 18 O in the paleosols ( Fig. 2b ). Therefore, the relationship between Se and δ 18 O in the interglacial time periods appears to reflect a dependence of Se on the precipitation input from the EASM. In contrast, in the loess layers we find only moderately weak relationships between Se and δ 18 O ( Supplementary Fig. 2a ), and between SMI and δ 18 O ( Supplementary Fig. 2b ). 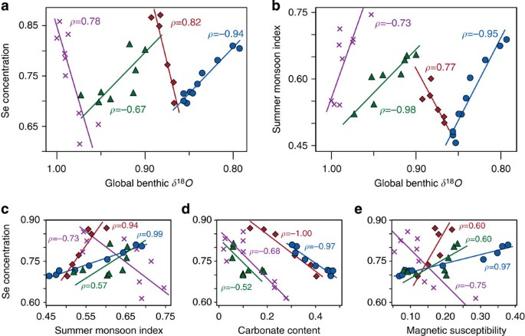Figure 2: Relationship between selenium and paleoclimate proxies in interglacial time periods. All data were smoothed and normalized (see Methods). Relationship between global benthicδ18O (ref.54) and (a) Se and (b) summer monsoon index (SMI)31and, correlation plots between Se and (c) summer monsoon index, (d) carbonate content and (e) magnetic susceptibility paleomonsoon proxies31. Time periods (blue circle—period I: 2.31–1.56 Ma, red diamond—period II: 1.50–1.29 Ma, green triangle—period III: 1.26–0.83 Ma, purple cross—period IV: 0.78–0.16 Ma) are based on the alternating positive and negative correlations between Se, SMI and global benthicδ18O seen inaandb. Rho (ρ) indicates Spearman’s correlation coefficient and trend lines in all panels are reduced major axis (RMA) regressions. Figure 2: Relationship between selenium and paleoclimate proxies in interglacial time periods. All data were smoothed and normalized (see Methods). Relationship between global benthic δ 18 O (ref. 54 ) and ( a ) Se and ( b ) summer monsoon index (SMI) [31] and, correlation plots between Se and ( c ) summer monsoon index, ( d ) carbonate content and ( e ) magnetic susceptibility paleomonsoon proxies [31] . Time periods (blue circle—period I: 2.31–1.56 Ma, red diamond—period II: 1.50–1.29 Ma, green triangle—period III: 1.26–0.83 Ma, purple cross—period IV: 0.78–0.16 Ma) are based on the alternating positive and negative correlations between Se, SMI and global benthic δ 18 O seen in a and b . Rho ( ρ ) indicates Spearman’s correlation coefficient and trend lines in all panels are reduced major axis (RMA) regressions. Full size image Se linked to monsoon proxies When examining the relationship between the effective precipitation (SMI) and Se in the four time periods, we found that the concentration of Se in the paleosols depends strongly on precipitation from the EASM over periods I and II (2.31–1.56 Ma and 1.50–1.29 Ma, Fig. 2c ). During these two periods, SMI ( Table 1 ) was weaker compared with the two more recent periods (periods III and IV, 1.26–0.83 Ma and 0.78–0.16 Ma). However, the strength of the EAWM, as recorded by mean quartz grain size and mass accumulation rates, was also lower during periods I and II ( Table 1 ), which indicates that the relationship between Se and the EASM is more apparent in times of lower dust input. Similar to other major components of global climate, EASM strength has fluctuated over orbital timescales [31] . Wavelet analyses (Methods, Supplementary Discussion and Supplementary Figs 3 and 4 ) reveal 100- and 400-kyr periods in the Se and SMI time series which are coincident with the eccentricity orbital forcing. These results provide further evidence for the relationship between Se and effective precipitation (that is, SMI). Table 1 Relative strength of East Asian summer monsoon and East Asian winter monsoon over time periods I–IV. Full size table Our results could imply two scenarios: (1) Se has been remobilized via leaching during pedogenesis, and/or (2) precipitation is a source of Se, in addition to Se present in the incoming dust. We begin by assessing the first scenario of potential Se remobilization via leaching. Leaching of calcium carbonate and re-deposition is a commonly observed phenomenon over the entire CLP [29] , which has resulted in the loss of carbonate from paleosols and an associated depletion of strontium (Sr) and other trace elements [37] . Indeed, we find a moderate positive correlation between Sr and carbonate content ( ρ =0.69, P <0.001) over all the interglacial periods. Therefore, we expect that a positive correlation between Se and the carbonate content would reveal any possible leaching and co-deposition of Se with carbonates. However, in the interglacial time periods I, II and IV, we find significant moderate-to-strong (period I: ρ =−0.97, P <0.001, period II: ρ =−1.00, P <0.001, and period IV: ρ =−0.68, P =0.004) negative correlation between Se and carbonate content ( Fig. 2d ) and a moderate but slightly less significant ( ρ =−0.52, P =0.180) negative correlation in period III ( Fig. 2d ), which suggests that while decalcification and leaching occurred, Se was not remobilized. Further support for the immobile behaviour of Se is provided by batch-leading experiments (Methods and Supplementary Table 1 ) which showed that the maximum amount of Se(IV) and Se(VI) that was leached during the experiments was always below the limit of detection for our ultra-trace pre-concentration speciation method [38] . In addition, principal component analysis (PCA) of geochemical and paleoclimate data (Methods, Supplementary Discussion and Supplementary Table 2 ) provides further evidence of the immobility of Se. In contrast to the loess–paleosol sequence, the underlying Red Clay formation (age ~6.8–2.6 Ma) is highly weathered and extensive carbonate leaching has been described in this formation [32] , [39] . In the late Miocene aged section of the Red Clay (6.8–5.3 Ma), the strong positive correlation between Se and carbonate ( ρ =0.85, P <0.001, Fig. 3a ) indicates that Se has leached and re-deposited with calcium carbonate. Therefore, the behaviour of Se in the older section of the Red Clay formation is opposite to the consistent immobile behaviour observed in the overlying paleosols. Further, there is a moderate negative correlation of Se with magnetic susceptibility ( Fig. 3b , late Miocene: ρ =−0.66, P =0.003 and Pliocene: ρ =−0.59, P <0.001) throughout the entire Red Clay leading to an overall moderate-to-strong negative correlation between SMI and Se ( Fig. 3c,d , late Miocene: ρ =−0.95, P <0.001 and Pliocene: ρ =−0.71, P <0.001). Because the relationship between Se and the EASM in the overlying paleosols does not appear to have been related to leaching processes, we suggest that the second scenario is valid and that precipitation is a source of Se. 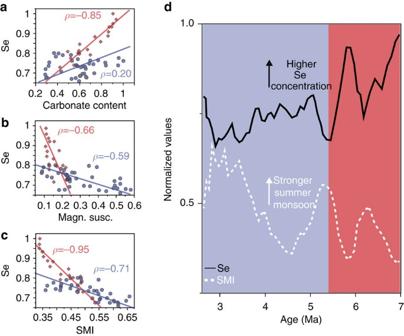Figure 3: Selenium and paleo-precipitation proxy trends in the Neogene red clay formation. Colours of symbols ina–crepresent the Miocene (red)-Pliocene (blue) epochs seen ind. All values shown are normalized. (a) Se versus carbonate content, (b) Se versus magnetic susceptibility, (c) Se versus summer monsoon index (SMI) and (d) time series of smoothed and normalized Se (black line) and SMI (dashed white line). Rho (ρ) indicates Spearman’s correlation coefficient and trend lines ina–care reduced major axis (RMA) regressions. Figure 3: Selenium and paleo-precipitation proxy trends in the Neogene red clay formation. Colours of symbols in a – c represent the Miocene (red)-Pliocene (blue) epochs seen in d . All values shown are normalized. ( a ) Se versus carbonate content, ( b ) Se versus magnetic susceptibility, ( c ) Se versus summer monsoon index (SMI) and ( d ) time series of smoothed and normalized Se (black line) and SMI (dashed white line). Rho ( ρ ) indicates Spearman’s correlation coefficient and trend lines in a – c are reduced major axis (RMA) regressions. Full size image Generally, in aerobic soil environments, the oxyanions Se(IV) and Se(VI) are the dominant species of Se. These oxyanions are known to form complexes with organic matter, and adsorb to Fe-oxyhydroxides and clay minerals [40] , [41] , [42] , [43] , [44] , [45] , [46] . Selenite has a similar affinity for sorption on haematite, goethite and amorphous ferric oxide [47] , and selenate has been found to form inner-sphere surface complexes on haematite and a mixture of inner- and outer-sphere surface complexes on goethite and hydrous ferric oxide [40] . Due to these interactions, soil chemistry (that is, pH, organic carbon content, clay content and so on) is a major factor in controlling Se retention in soils. Because there is no evidence of persistent reducing conditions in the loess–paleosol sequences and it is known that Se being deposited from the atmosphere is largely in the form of Se(IV) and Se(VI) [17] , we expect that oxidized Se species are dominant in the loess–paleosol sequences. Additionally, it is known that paedogenesis of the loess material leads to increases in organic carbon content and to the formation of secondary Fe-oxyhydroxides and clay minerals [29] that could all potentially provide binding sites for Se species. Therefore, we have evaluated how organic carbon, Fe-oxyhydroxides and clay minerals may interact with these oxidized Se species. We found no indication that Se sequestration by organic carbon is a major controlling factor of the Se distribution within the paleosols, since the amounts of organic carbon in paleosols are relatively low (0.03–0.62 wt%, Supplementary Table 3 ) and characterized by a moderate negative ( ρ =−0.59, P =0.0003) correlation with Se. In contrast, the similar correlations between SMI and Se, and magnetic susceptibility and Se (see Fig. 2c,e ) suggest that secondary ferrimagnetic minerals provide sorption sites for Se species. However, when we consider the negative relationship between Se and magnetic susceptibility for period IV (0.78–0.16 Ma, Fig. 2c ), this explanation does not work, especially considering that during this period the magnetic susceptibility and the inferred EASM strength was higher than in previous times [31] , [48] (also see Table 1 ). Therefore, in time period IV, Se may possibly be related to Fe-bearing clay minerals or non-magnetic or less-magnetic Fe minerals such as haematite and goethite which are ~10 times more abundant in the paleosol than the more magnetic magnetite and maghemite phases [21] . X-ray absorption spectroscopy (XAS) performed on nine samples at the Fe K-edge (see Methods, Supplementary Discussion , Supplementary Fig. 5 and Supplementary Table 4 ) suggested that the largest fraction of Fe (at least 50% and up to 80%) was contained in phyllosilicate clay minerals. Both illite and smectite clays have been shown to be strong sorbents of Se [44] and indeed we observe similar trends between these Fe-bearing clay mineral abundances and Se concentrations in the Lingtai section ( Supplementary Fig. 6 ). This observation suggests that clay minerals play a role in the adsorption of Se, especially in the youngest part of the section (period IV, 0.78–0.16 Ma). Nevertheless, further and more in-depth investigations are required to quantitatively and qualitatively assess the mineralogical controls on Se sorption in the CLP. Our results suggest that EASM-derived precipitation is a source of Se in the CLP. This finding may help to explain the similarity between precipitation patterns and soil Se patterns in the area of China south of the summer monsoon limit ( Fig. 1a,b ); however, future work should investigate this further. Because the Se-poor belt stretching across China is at the edge of both the EASM and the EAWM, we suggest that the Se-deficient soils in this region are related to limited atmospheric Se input via both wet and dry deposition. Annual precipitation trends in China are forecasted to change drastically in the coming decades [49] , and these changes could thus have important implications for future Se distribution throughout China. Furthermore, anthropogenic Se emissions from activities such as coal combustion and metallurgy are already an important component of the total atmospheric Se budget [12] , [13] , [14] and can be expected to increase in the future. With China’s continued rapid economic growth and a 1.9% average annual increase in coal combustion predicted through 2040 (ref. 50 ), anthropogenic Se emissions will need to be considered in future assessments of the terrestrial distribution of Se in China. We suggest that low atmospheric Se inputs could play an important role in explaining widespread low-Se environments in other inland regions of the world. Future work should focus on refining our understanding of the role of climate on atmospheric Se deposition not only within China but globally, as such knowledge will pave the way for predictions of terrestrial Se distributions, which will help to prevent health hazards related to Se deficiency. Geochemical analyses Air-dried loess and paleosol samples ( n =137) were crushed and homogenized with an agate mortar and pestle. Aliquots (50 mg) of sample were mixed in Teflon vessels with 4 ml 69% HNO 3 and 1 ml 30% H 2 O 2 and digested at 180 °C and 3.75 bar for 25 min in a microwave digestion unit. The digestions were diluted with deionized H 2 O and analysed using an inductively coupled plasma mass spectrometry with gas collision cell. Repeat analyses of NIST RM-8704 Buffalo River sediment standard (BRS-STD), IAG QC-13 loess quality-control material and duplicate sample digestions gave results with generally <10% relative standard deviation (RSD), and <5% RSD for all elements considered in this study. For Se analyses, 200 mg of sample were mixed in Teflon beakers with 3:1 HCl (32%):HNO 3 (69%) and digested on a hot plate at 120 °C. The digestions were diluted 1:10 with deionized H 2 O. In total, 10 ml of diluted samples were mixed with 15 ml of 32% HCl and were reduced in closed vessels at 100 °C for 30 min in the microwave. Samples were diluted and analysed using an hydride generation atomic fluorescence spectrometry. Analysis of JT Baker Se standard and repeat digestions of Buffalo River sediment and 15 samples yielded results with a precision of ≤7% RSD (excluding one outlier, LT-15156, 67% RSD), and an average recovery rate of 85% calculated from BRS-STD. A procedural blank was analysed with each set of digestions and the resulting concentration was subtracted from the determined Se concentration. Procedural blanks averaged 5.6 ng l −1 . Total carbon was analysed with a CHNS-O elemental analyzer using 5–10 mg of sample. Analysis of a reference soil material (Hekatech Soil Standard HE33860401) and duplicate samples yielded precision of <8% RSD. For inorganic carbon, 5–10 mg of sample was analysed using a carbon coulometer. Analysis of a carbonate standard reference material (Merck) and duplicate samples yielded precisions of ≤ 1% RSD, except for one sample (LT-7300, 18.6% RSD), which was below the detection limit of the instrument (0.01 μg total carbon). The organic carbon content was calculated as the difference between the total and inorganic carbon ( Supplementary Table 3 ). Fe K-edge XAS Fe K-edge XAS was used to study the speciation of Fe in three loess, three paleosol and three red clay samples. The samples were thoroughly mixed with cellulose and pressed into 13-mm pellets for analysis in transmission mode at room temperature. The XAS data were collected at the Swiss Norwegian Beamline (SNBL, extended X-ray absorption fine structure (EXAFS) station BM01B) at the European Synchrotron Radiation Facility (Grenoble, France). A Si(111) double-crystal monochromator was used for beam energy selection and ionization chambers to record the incident and transmitted photon intensity. Beam energy was calibrated by setting the first maximum of the first derivative of the absorption edge of a metallic Fe foil to 7,112 eV. For each sample, four scans (12 min each) were collected and averaged. The X-ray absorption near-edge structure and EXAFS spectra were extracted using the software code Athena [51] . The E 0 was fixed at 7,128.5 eV. The spectra were normalized by subtracting a first-order polynomial fitted to the data from −100 to −30 eV before the edge and subsequently dividing through a second-order polynomial fitted to the data from 60 to 450 eV above the edge. EXAFS spectra were extracted using the Autobk algorithm ( R bkg =0.9; k -weight=3, spline k -range 0–11.8 Å −1 ). The k 3 -weighted EXAFS spectra were analysed by linear combination fitting over the k -range 2–11 Å −1 using software from beamline 10.3.2 at the Advanced Light Source (Berkeley, USA) [52] . Linear combination fitting analysis was based on a collection of own and published reference spectra. Starting with the best one-component fit, the number of components was increased as long as the normalized sum of the squared residuals (NSSR=∑(data i –fit i ) 2 /∑(data i ) 2 ) of the best n +1-component fit was at least 10% lower than the NSSR of the best n -component fit. Se-leaching tests In order to assess the potential mobility of Se during weathering and paedogenesis, we carried out leaching experiments following the method described in Lenz et al. [38] This method is based on pre-concentration of the analytes, followed by chromatographic separation and element specific (inductively coupled plasma mass spectrometry) detection and has been successfully used to quantify Se leached from strongly Se-depleted volcanic ashes (<0.05 mg kg −1 Se). Briefly, ~500 mg of loess/paleosol sample was leached in test tubes with ~12.5 ml ultrapure deionized water (sediment:water ratio of ~1:25) for 1.5 h on a shaking plate. The samples were centrifuged (21,500 g , 10 min) and the supernatant was filtered and analysed for Se speciation. Neither Se(IV) nor Se(VI) was detected in any sample (the limit of detection being 3 σ of blank baselines at the Se(IV)/Se(VI) retention times). For the sample lowest in Se content (LT-16156), this corresponded to a maximal amount of 5.8% and 11.5% that could have leached as Se(IV) and Se(VI), respectively, without being detected. Additionally, duplicate leaches of a Chinese loess standard reference material (GBW07408 GSS-8) with a Se concentration of 0.10±0.01 mg kg −1 also had Se leachate concentrations below the LOD. Statistical analysis of trace element and proxy data All data were analysed using JMP 10.0 statistical software ( http://www.jmp.com/support/downloads/pdf/jmp1001/using_jmp.pdf ), except for reduced major axis regression lines which were calculated using lmodel2 package in R statistical software ( http://www.r-project.org/ ). For comparisons with paleomonsoon proxies [31] and global benthic δ 18 O records [53] (see Fig. 2 in main text), red clay, paleosol and loess samples were separated into groups, data were smoothed using a five-point moving average and values were normalized with respect to the maximum value. Wavelet analysis In order to assess the strength of correlation between the SMI and Se in frequency domain, we have carried out wavelet analysis after linear interpolation of the two time series and compared the individual continuous wavelet transforms using wavelet coherency analysis. The average time resolution of our data is ~50 kyr and therefore any periodicities that lie in the 41- and 23-kyr orbital domain will not be captured by our analysis. The wavelet and wavelet coherence analyses were carried out using the script provided by Grinsted et al. [54] , which is an expanded wavelet analysis toolkit based on the work of Torrence and Compo [55] . PCA PCA was carried out in JMP to understand groupings of the analysed elements and paleomonsoon proxies. All elements from inductively coupled plasma mass spectrometry and hydride generation atomic fluorescence spectrometry analyses (Al, Fe, Mg, Ca, Mn, V, Cr, Co, Ni, Cu, Zn, As, Sr, Cd, Pb and Se), winter monsoon proxies (mean quartz grain size, mean bulk grain size, dust mass accumulation rate) and summer monsoon proxies (magnetic susceptibility, carbonate content and SMI) were used in the PCA analysis. The JMP software package calculates each principal component by taking a linear combination of an eigenvector of the correlation matrix with a variable. Similar to our other data analysis, we have separated data into loess, paleosol and red clay groups. How to cite this article: Blazina, T. et al. Terrestrial selenium distribution in China is potentially linked to monsoonal climate. Nat. Commun. 5:4717 doi: 10.1038/ncomms5717 (2014).